Reconstitution of microtubule into GTP-responsive nanocapsules Nanocapsules that collapse in response to guanosine triphosphate (GTP) have the potential as drug carriers for efficiently curing diseases caused by cancer and RNA viruses because GTP is present at high levels in such diseased cells and tissues. However, known GTP-responsive carriers also respond to adenosine triphosphate (ATP), which is abundant in normal cells as well. Here, we report the elaborate reconstitution of microtubule into a nanocapsule that selectively responds to GTP. When the tubulin monomer from microtubule is incubated at 37 °C with a mixture of GTP (17 mol%) and nonhydrolysable GTP* (83 mol%), a tubulin nanosheet forms. Upon addition of photoreactive molecular glue to the resulting dispersion, the nanosheet is transformed into a nanocapsule. Cell death results when a doxorubicin-containing nanocapsule, after photochemically crosslinked for properly stabilizing its shell, is taken up into cancer cells that overexpress GTP. An ideal nanocarrier for drug delivery would be the one that can selectively collapse to release preloaded drugs in response to endogenous reporters overexpressed in disease tissues [1] , [2] , [3] , [4] , [5] , [6] , [7] , [8] , [9] . Since adenosine triphosphate (ATP) is known to be present at high levels in cancer tissues [10] , ATP-responsive nanocarriers might be a promising candidate [3] , [4] , [5] , [6] , [7] . In 2013, using partially modified biomolecular machine chaperonin GroEL as a monomer, we succeeded in developing a one-dimensional supramolecular polymer that can be depolymerized by the action of ATP to release its cargo [3] . However, ATP is also present in normal cells at rather high concentrations (>1 mM) [11] , and thus disease-selective drug delivery using ATP as the endogenous reporter cannot always be ensured. In the present work, we developed a nanocarrier ( CL NC GTP/GTP* ; Fig. 1e ) that selectively responds to guanosine triphosphate (GTP). GTP is an intracellular molecule involved in many essential biological processes [12] , [13] , [14] , [15] , [16] , [17] , [18] , [19] , [20] , [21] , [22] , [23] , [24] , [25] , such as cell division [12] , nucleotide synthesis [13] , and cell signaling [14] . In the cell division process, the tubulin heterodimer (THD), which constitutes microtubules (MTs), uses GTP as an energy source to induce its polymerization and depolymerization [15] , [16] , [17] , [18] , [19] , [20] . GTP is also used as a component for the self-replication of RNA viruses [26] , [27] , [28] , [29] such as coronaviruses. Notably, GTP is abundant in certain diseased cells (1.5–4.5 mM) [30] such as rapidly proliferating cancer cells [31] and RNA virus-infected cells [32] , whereas the concentration of GTP, unlike that of ATP, is negligibly low in normal cells (<0.3 mM) [33] . Therefore, GTP-responsive nanocarriers have the great potential to efficiently cure cancer and RNA virus-induced diseases including coronavirus disease 2019 (COVID-19) [29] . Although GTP-responsive carriers have already been reported, those carriers also respond to ATP [5] . So far, nanocarriers capable of responding solely to GTP have never been reported. Fig. 1: Strategy used to prepare THD-based GTP-responsive CL NC GTP/GTP* . a Schematic illustrations of tubulin heterodimers (THDs) hybridized with GTP (THD GTP ), its nonhydrolysable analogue GTP* (THD GTP* ), and GDP (THD GDP ) at its β -tubulin unit. b Schematic illustration of two self-assembling modes of THD into microtubules (MTs). MT GTP depolymerizes into THD GDP upon GTP hydrolysis. THD GDP rehybridizes with GTP after a GTP treatment, facilitating the formation of MT GTP . In contrast, MT GTP* does not undergo depolymerization. c Molecular structures of photoreactive molecular glues ( \({{{\mathrm{Glue}}}}^{{{{\mathrm{CO}}}}_2-}\) , \({{{\mathrm{Glue}}}}^{{{{{\mathrm{CO}}}}_{2}-}{\mathrm {Me}}}\) , and Glue FITC ) bearing three guanidinium ions (Gu + ) and benzophenone (BP) groups at their periphery and \({{{{\mathrm{CO}}}}_2-}\) , CO 2 Me, and FITC groups at the focal core. d The molecular glue covalently binds to the protein surface at its photoexcited BP groups after the noncovalent adhesion via a Gu + /oxyanion multivalent salt-bridge interaction. e Schematic illustration of the multistep procedure for the synthesis of crosslinked nanocapsules ( CL NC GTP/GTP* ) from MT GTP . MT GTP is depolymerized into THD GDP , which is incubated with a mixture of GTP* (83 mol%) and GTP (17 mol%) to form nanosheet NS GTP/GTP* . Upon treatment with \({{{\mathrm{Glue}}}}^{{{{\mathrm{CO}}}}_2-}\) , NS GTP/GTP* is transformed into spherical nanocapsules (NC GTP/GTP* ), which are further exposed to UV light, affording CL NC GTP/GTP* . Upon addition of GTP, CL NC GTP/GTP* collapses through the conformational change of the THD units induced by GTP hydrolysis. Full size image The nanocapsule (NC) that selectively responds to GTP to release a preloaded drug consists of THD. As shown in Fig. 1a , THD is composed of α -tubulin (green) and β -tubulin (cream), both of which bind to GTP. Notably, GTP attached to the α -tubulin unit is neither hydrolysable into GDP nor replaceable with other nucleoside phosphates. In contrast, GTP attached to the β -tubulin unit is known to be hydrolysable to GDP, which can be replaced with, e.g., GTP*, a nonhydrolysable GTP analogue (guanylyl 5’- α , β -methylenediphosphonate), affording THD GTP* (for convenience, only variable nucleoside phosphates attached to the β -tubulin unit are shown as a subscript). Both THD GTP and THD GTP* , when heated at 37 °C, have been reported to self-assemble into microtubules MT GTP and MT GTP* , respectively (Fig. 1b ) [34] , [35] . Although MT GTP depolymerizes into THD GDP synchronously with the hydrolysis of hybridized GTP to GDP, MT GTP* does not depolymerize into THD GDP* because of the nonhydrolysable nature of GTP*. Therefore, our original motivation was to tackle a challenge of modulating the stability of MTs against depolymerization by changing the THD GTP /THD GTP* molar ratio. However, we unexpectedly found that the coassembly of THD GTP and THD GTP* at a certain mixing molar ratio resulted in the formation of a leaf-like 2D nanosheet (NS) rather than MT (Fig. 1e ). Because of the increasing importance of 2D objects [36] , [37] , this finding prompted us to functionalize NS using the molecular glue technology [38] , [39] , [40] , which we developed for noncovalently functionalizing biomolecules such as proteins, nucleic acids, and phospholipid membranes, and also inorganic materials. Molecular glues are designed to carry multiple guanidinium ion (Gu + ) groups and strongly adhere to such biomolecules under physiological conditions by taking advantage of a multivalent salt-bridge interaction with their oxyanionic functionalities (Fig. 1d ). For this purpose, we chose \({{{\mathrm{Glue}}}}^{{{{\mathrm{CO}}}}_2-}\) (Fig. 1c ) and incubated it with NS. To our surprise, NS was transformed into a spherical nanocapsule NC (Fig. 1e ). Using its photochemically modified version ( CL NC GTP/GTP* ; Fig. 1e ), we successfully encapsulated and delivered doxorubicin (DOX) [41] , an anticancer drug, into GTP-overexpressing cancer cells to cause cell death. 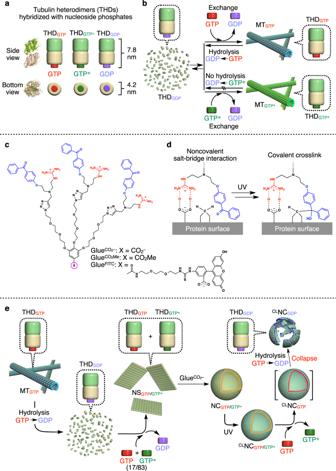Fig. 1: Strategy used to prepare THD-based GTP-responsiveCLNCGTP/GTP*. aSchematic illustrations of tubulin heterodimers (THDs) hybridized with GTP (THDGTP), its nonhydrolysable analogue GTP* (THDGTP*), and GDP (THDGDP) at itsβ-tubulin unit.bSchematic illustration of two self-assembling modes of THD into microtubules (MTs). MTGTPdepolymerizes into THDGDPupon GTP hydrolysis. THDGDPrehybridizes with GTP after a GTP treatment, facilitating the formation of MTGTP. In contrast, MTGTP*does not undergo depolymerization.cMolecular structures of photoreactive molecular glues (\({{{\mathrm{Glue}}}}^{{{{\mathrm{CO}}}}_2-}\),\({{{\mathrm{Glue}}}}^{{{{{\mathrm{CO}}}}_{2}-}{\mathrm {Me}}}\), and GlueFITC) bearing three guanidinium ions (Gu+) and benzophenone (BP) groups at their periphery and\({{{{\mathrm{CO}}}}_2-}\), CO2Me, and FITC groups at the focal core.dThe molecular glue covalently binds to the protein surface at its photoexcited BP groups after the noncovalent adhesion via a Gu+/oxyanion multivalent salt-bridge interaction.eSchematic illustration of the multistep procedure for the synthesis of crosslinked nanocapsules (CLNCGTP/GTP*) from MTGTP. MTGTPis depolymerized into THDGDP, which is incubated with a mixture of GTP* (83 mol%) and GTP (17 mol%) to form nanosheet NSGTP/GTP*. Upon treatment with\({{{\mathrm{Glue}}}}^{{{{\mathrm{CO}}}}_2-}\), NSGTP/GTP*is transformed into spherical nanocapsules (NCGTP/GTP*), which are further exposed to UV light, affordingCLNCGTP/GTP*. Upon addition of GTP,CLNCGTP/GTP*collapses through the conformational change of the THD units induced by GTP hydrolysis. Reconstitution of MT GTP into NC GTP/GTP* Figure 1e illustrates the overall procedure for the synthesis of NC GTP/GTP* from microtubule MT GTP . As a typical example of the procedure depicted in the flow chart in Fig. 2a , a 1,4-piperazinediethanesulfonic acid (PIPES) buffer (pH 6.8) solution of MT GTP (5.8 mg ml –1 , Fig. 2c ) was cooled at 4 °C, whereupon MT GTP underwent complete depolymerization within 3 h to yield THD GDP quantitatively (Fig. 2d ) [42] . As observed by dynamic light scattering (DLS), the characteristic polydisperse feature of one-dimensional (1D) MT GTP (Fig. 2b , gray) changed to a monodisperse feature with a reduced hydrodynamic diameter of 8 nm (Fig. 2b , blue). Then, THD GDP (0.3 mg ml –1 ) was immersed in a PIPES buffer solution of a mixture of GTP and GTP* (300 µM in total) with a GTP* content of 83 mol% at 37 °C for 30 min. 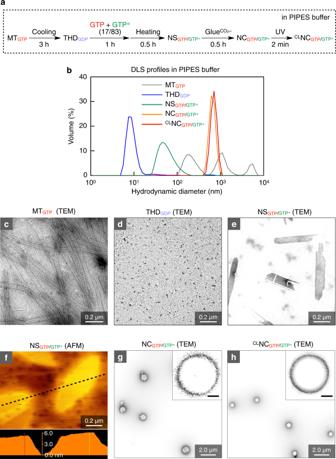Fig. 2: Reconstitution of MT intoCLNCGTP/GTP*. aA typical synthetic procedure for the preparation ofCLNCGTP/GTP*.bDLS profiles of MTGTP(gray), THDGDP(blue), NSGTP/GTP*(green), NCGTP/GTP*(orange), andCLNCGTP/GTP*(red) in PIPES buffer.c–eTEM images of MTGTP(5.8 mg ml–1;c), THDGDP(0.3 mg ml–1;d), and NSGTP/GTP*(0.3 mg ml–1;e).fAFM image of NSGTP/GTP*(0.3 mg ml–1) and its height profile.g,hTEM images of NCGTP/GTP*(13 µg ml–1;g) andCLNCGTP/GTP*(13 µg ml–1;h). All TEM samples were negatively stained with uranyl acetate. Inset scale bars, 250 nm. Under the present conditions, THD GDP was converted via the exchange events of GDP → GTP and GDP → GTP* into a mixture of THD GTP and THD GTP* , which then spontaneously coassembled into NS GTP/GTP* (Fig. 2e ). The small-angle X-ray scattering (SAXS) profile of NS GTP/GTP* showed that its scattering intensity was proportional to q –2 in a small q region, which is characteristic of two-dimensional (2D) structures (Supplementary Fig. 9 ). As determined by atomic force microscopy (AFM), the average thickness of leaf-like NS GTP/GTP* was 5 nm (Fig. 2f ). Here, the content of GTP* in the mixture of GTP and GTP* employed for the assembly of THD GDP was critical for its successful transformation into NS GTP/GTP* . When the content of GTP* ranged from 85–100 mol%, THD preferentially assembled into MT rather than NS (Supplementary Fig. 10 ), whereas THD barely assembled when its GTP* content was in the range of 0–70 mol% (Supplementary Fig. 11 ). Namely, the optimum THD GTP /THD GTP* molar ratio for the coassembly into NS is narrow, roughly with a GTP* content of 70–85 mol%. By means of nuclear magnetic resonance (NMR) spectroscopy in DMSO, NS GTP/GTP* prepared at a GTP* content of 83 mol% was found to contain 65 mol% of THD GTP* (Supplementary Fig. 12 ). It is known that MT GTP and MT GTP* , prepared from THD GTP and THD GTP* , respectively, are formed by edge-closing of NS GTP and NS GTP* as transient precursors [43] . Note that the longer axis of THD GTP is shorter than that of THD GTP* [44] . We suppose that this mismatch possibly affords unfolded NS GTP/GTP* rather than folded MT GTP/GTP* . Indeed, when THD GTP* (GTP* content of 83 mol%) was coassembled with THD GTPγS (THD hybridized with guanosine 5’-O-(3-thiotriphosphate), GTPγS), whose length is likewise shorter than THD GTP* [44] , NS GTPγS/GTP* was formed (Supplementary Fig. 13 ), whereas the coassembly of THD GTP and THD GTPγS (GTPγS content of 83 mol%), whose longer axes are close in length to each other [44] , resulted in MT GTP/GTPγS (Supplementary Fig. 14 ). NS GTP/GTP* was transformed into NC GTP/GTP* when it was incubated with Glue CO– (100 µM) in PIPES buffer at 37 °C for 30 min (Fig. 1e ). This anomalous transformation was accompanied by a large change in the hydrodynamic diameter from 65 nm (Fig. 2b , green) to 660 nm (Fig. 2b , orange) with a slight increase in the zeta potential from –42.2 to –39.0 mV. Transmission electron microscopy (TEM) showed that the newly formed object NC GTP/GTP* was a hollow sphere (Fig. 2g ). When MT GTP* and THD GDP instead of NS GTP/GTP* were likewise treated with \({{{\mathrm{Glue}}}}^{{{{\mathrm{CO}}}}_2-}\) , ill-defined agglomerates resulted (Supplementary Figs. 15 and 16 ). Fig. 2: Reconstitution of MT into CL NC GTP/GTP* . a A typical synthetic procedure for the preparation of CL NC GTP/GTP* . b DLS profiles of MT GTP (gray), THD GDP (blue), NS GTP/GTP* (green), NC GTP/GTP* (orange), and CL NC GTP/GTP* (red) in PIPES buffer. c – e TEM images of MT GTP (5.8 mg ml –1 ; c ), THD GDP (0.3 mg ml –1 ; d ), and NS GTP/GTP* (0.3 mg ml –1 ; e ). f AFM image of NS GTP/GTP* (0.3 mg ml –1 ) and its height profile. g , h TEM images of NC GTP/GTP* (13 µg ml –1 ; g ) and CL NC GTP/GTP* (13 µg ml –1 ; h ). All TEM samples were negatively stained with uranyl acetate. Inset scale bars, 250 nm. Full size image Photochemical crosslinking of NC GTP/GTP* The physical stability of NC GTP/GTP* is important for its utilization as a carrier for drug delivery. Through several different experiments, we noticed that NC GTP/GTP* immediately collapsed upon incubation with albumin or serum in buffer, indicating its insufficient stability as a drug carrier. Here, we would like to point out a great advantage of \({{{\mathrm{Glue}}}}^{{{{\mathrm{CO}}}}_2-}\) and its homologues that their multiple benzophenone (BP) groups upon photoexcitation enable covalent crosslinking with adhering proteins (Fig. 1d ). Successful examples so far reported include microtubule and kinesin [39] , whose dynamic behaviors could be attenuated by the reaction with photoexcited molecular glues. In the present work, by using fluorescent FITC-appended Glue FITC (Fig. 1c , FITC; fluorescein isothiocyanate) derived from \({{{\mathrm{Glue}}}}^{{{{\mathrm{CO}}}}_2-}\) , we first confirmed that \({{{\mathrm{Glue}}}}^{{{{\mathrm{CO}}}}_2-}\) has a sufficient photoreactivity with the constituent (THD) of NC GTP/GTP* . As shown in Supplementary Fig. 17 , the reaction mixture, after being exposed to UV light (300 nm) in PIPES buffer, showed the presence of a fluorescence-emissive covalent adduct between THD GDP and Glue FITC in sodium dodecyl sulfate polyacrylamide gel electrophoresis (SDS-PAGE). Then, we investigated whether this photochemical approach can provide NC GTP/GTP* with a sufficient physical stability by crosslinking the shell. Thus, a PIPES buffer solution of NC GTP/GTP* was exposed to UV light for 2 min, where TEM (Fig. 2h ) and AFM imaging results (Supplementary Fig. 18 ) and DLS profiles (Fig. 2b , red) showed that crosslinked (CL) CL NC GTP/GTP* was spherical and remained intact even upon incubation with albumin (0.1 mg ml –1 ) or serum (0.01%) (Supplementary Figs. 19 and 20 ). CL NC GTP/GTP* , when prepared using Glue FITC instead of \({{{\mathrm{Glue}}}}^{{{{\mathrm{CO}}}}_2-}\) , was fluorescent (Supplementary Fig. 21 ), indicating the presence of the molecular glue in CL NC GTP/GTP* . Computational simulation of the assembly of NS GTP/GTP* Considering that tubulin nanosheets NS GTP/GTP* are, on average, 0.04 µm 2 wide and 4.2 nm thick, the formation of NC GTP/GTP* (surface area; ~6.2 µm 2 , membrane thickness; 50 nm) requires at least 1000 pieces of NS GTP/GTP* to assemble. Note that \({{{\mathrm{Glue}}}}^{{{{\mathrm{CO}}}}_2-}\) carrying both Gu + and \({{{{\mathrm{CO}}}}_2-}\) groups in its structure can self-assemble via their salt-bridge interaction. In the initial stage of the transformation of NS GTP/GTP* into NC GTP/GTP* , we postulate that a certain number of \({{{\mathrm{Glue}}}}^{{{{\mathrm{CO}}}}_2-}\) molecules utilize their Gu + groups to form a salt-bridged network with the surface \({{{{\mathrm{CO}}}}_2-}\) groups on NS GTP/GTP* (Fig. 1d ) as well as the focal-core CO 2 – group in \({{{\mathrm{Glue}}}}^{{{{\mathrm{CO}}}}_2-}\) . This adhesion event can lower the surface charge density of NS GTP/GTP* and enhance its hydrophobic stacking, which is secured by possible reorganization of the salt-bridged polymeric networks on NS GTP/GTP* (Fig. 1e ). We performed all atom molecular dynamics (MD) simulations [45] to explore the adhesion of \({{{\mathrm{Glue}}}}^{{{{\mathrm{CO}}}}_2-}\) and the effect of this event on the tubulin assembly. From a full MT model (PDB code: 3J6E), we obtained its partial structure composed of three laterally assembled THD GTP* units ([THD GTP* ] 3 ) as a model of NS (Fig. 3a ). The MD simulation suggested that \({{{\mathrm{Glue}}}}^{{{{\mathrm{CO}}}}_2-}\) adopts a globular conformation in aqueous media with a hydrodynamic diameter of 1.5 nm (Fig. 3b , Supplementary Fig. 22 ). When exposed to 30 equivalents of \({{{\mathrm{Glue}}}}^{{{{\mathrm{CO}}}}_2-}\) (Fig. 3c , d ), [THD GTP* ] 3 enhances its hydrophobic nature (Fig. 3e , f ) as a result of the surface charge neutralization by adhering \({{{\mathrm{Glue}}}}^{{{{\mathrm{CO}}}}_2-}\) . In the solvent-accessible surface area of [THD GTP* ] 3 , the hydrophobic dominancy increases from 48% to 57% (Fig. 3g ). Notably, when \({{{\mathrm{Glue}}}}^{{{{\mathrm{CO}}}}_2-}\) was allowed to adhere onto [THD GTP* ] 3 , the molecular simulations suggested that [THD GTP* ] 3 adopts a slightly more flattened conformation, characterized by a distribution angle with an average value of ~156° (Fig. 3h, i , blue), compared with that of native [THD GTP* ] 3 (red). The simulations also showed that, even after the \({{{\mathrm{Glue}}}}^{{{{\mathrm{CO}}}}_2-}\) adhesion, [THD GTP* ] 3 preserved a certain level of flexibility (Fig. 3i ). We also calculated radial distribution functions g(r) between the charged groups of \({{{\mathrm{Glue}}}}^{{{{\mathrm{CO}}}}_2-}\) and the amino acid residues of [THD GTP* ] 3 . Supposedly, the CO 2 – groups in aspartic acid and glutamic acid are interactive with the Gu + groups in \({{{\mathrm{Glue}}}}^{{{{\mathrm{CO}}}}_2-}\) , while the cationic groups in lysine and arginine are interactive with the focal \({{{{\mathrm{CO}}}}_2-}\) group in \({{{\mathrm{Glue}}}}^{{{{\mathrm{CO}}}}_2-}\) . As expected, the g(r) data revealed that the Gu + groups in \({{{\mathrm{Glue}}}}^{{{{\mathrm{CO}}}}_2-}\) are largely populated near the \({{{{\mathrm{CO}}}}_2-}\) groups on the [THD GTP* ] 3 surface (Fig. 3j , blue), whereas they are scarcely populated around the polar but nonionic hydroxyl groups in serine, threonine, and tyrosine (Fig. 3j , gray). Meanwhile, the focal CO 2 – group in \({{{\mathrm{Glue}}}}^{{{{\mathrm{CO}}}}_2-}\) is not populated around the cationic groups on the [THD GTP* ] 3 surface (Supplementary Fig. 23 ). The computational calculation also showed that multiple adhering \({{{\mathrm{Glue}}}}^{{{{\mathrm{CO}}}}_2-}\) molecules can interact and self-assemble via a salt-bridge interaction between their Gu + and CO 2 – groups (Fig. 3j , red), which results in forming a dense Gu + /CO 2 – salt-bridged polymeric network on the [THD GTP* ] 3 surface (Fig. 3k ). This may promote the self-assembly of flexible NS GTP/GTP and stabilize them in the gently curved multilayered configuration of NC GTP/GTP* , as observed experimentally [46] , [47] . As a control experiment, the use of \({{{\mathrm{Glue}}}}^{{{{{\mathrm{CO}}}}_{2}-}{\mathrm {Me}}}\) (Fig. 1c ) having a focal ester group instead of its ionized form for the transformation of NS GTP/GTP* into NC GTP/GTP* resulted in an ill-defined agglomerate (Supplementary Fig. 24 ). Fig. 3: MD simulation of the adhesion events of Glue CO2– onto the surface of THD GTP* . a Three laterally assembled THD GTP* units ([THD GTP* ] 3 ) in MT GTP* as a partial model of NS. b An equilibrated MD snapshot of \({{{\mathrm{Glue}}}}^{{{{\mathrm{CO}}}}_2-}\) . c , d The outer ( c ) and inner ( d ) views of [THD GTP* ] 3 hybridized with 30 equivalents of \({{{\mathrm{Glue}}}}^{{{{\mathrm{CO}}}}_2-}\) . e , f The outer ( e ) and inner ( f ) views of [THD GTP* ] 3 with its electrostatic surface potential in the absence (upper) and presence (lower) of 30 equivalents of hybridized \({{{\mathrm{Glue}}}}^{{{{\mathrm{CO}}}}_2-}\) . Negative and positive potential areas are colored in red and blue, respectively. g The percentage of hydrophobic solvent-accessible surface area in the absence (47.5 ± 0.5; red) and presence (56.7 ± 2.0; blue) of 30 equivalents of hybridized \({{{\mathrm{Glue}}}}^{{{{\mathrm{CO}}}}_2-}\) . Bars represent mean values ± SD from 2000 data points. h , i [THD GTP* ] 3 observed from the top view ( h ) and its angle distributions ( i ) in the absence (red) and presence (blue) of 30 equivalents of hybridized \({{{\mathrm{Glue}}}}^{{{{\mathrm{CO}}}}_2-}\) . j Radial distribution functions g(r) of the Gu + groups in \({{{\mathrm{Glue}}}}^{{{{\mathrm{CO}}}}_2-}\) with carboxylates (blue) and non-ionic hydroxyl groups (gray) on the [THD GTP* ] 3 surface, and the carboxylate at the focal core of \({{{\mathrm{Glue}}}}^{{{{\mathrm{CO}}}}_2-}\) (red). k Schematic illustration of a possible adhesion event of \({{{\mathrm{Glue}}}}^{{{{\mathrm{CO}}}}_2-}\) onto NS GTP/GTP* and its effects on the features of NS GTP/GTP* . The Gu + groups in \({{{\mathrm{Glue}}}}^{{{{\mathrm{CO}}}}_2-}\) form a salt bridge with carboxylates on the NS GTP/GTP* surface and at the focal core of \({{{\mathrm{Glue}}}}^{{{{\mathrm{CO}}}}_2-}\) , and the \({{{\mathrm{Glue}}}}^{{{{\mathrm{CO}}}}_2-}\) -based polymeric network thus formed through this process increases the hydrophobicity of the NS GTP/GTP* surface, making NS GTP/GTP* more flatten. Full size image GTP-responsiveness of CL NC GTP/GTP* We investigated whether photochemically stabilized CL NC GTP/GTP* is responsive to GTP or not. Notably, the concentrations of both extracellular and intracellular GTP are lower than 0.3 mM in normal cells [33] . However, as already described in the introductory part, rapidly proliferating cancer cells and RNA virus-infected cells contain GTP in a concentration range of 1.5–4.5 mM [30] . Therefore, drug-loaded CL NC GTP/GTP* , when taken up into such GTP-rich environments, might selectively collapse to release its preloaded guest. Upon incubation for 100 min at 37 °C in PIPES buffer with 0.2 mM GTP, CL NC GTP/GTP* still maintained its spherical shape, as observed by TEM (Fig. 4a ). However, when the GTP concentration was increased to 0.5 mM, CL NC GTP/GTP* gradually collapsed (Fig. 4b ), displaying a polydisperse DLS profile in 100 min (Fig. 4c , green). This minimum concentration threshold is important for achieving the error-free delivery to GTP-enriched sites. We added Biomol Green TM as a phosphoric acid (PO 4 – ) detector to a mixture of CL NC GTP/GTP* and GTP (1 mM), and successfully detected PO 4 – by means of electronic absorption spectroscopy, indicating that CL NC GTP/GTP* has a GTPase activity (Fig. 4d ). Although THD GTP* , the constituent of CL NC GTP/GTP* , has no GTPase activity, the product upon incubation of THD GTP* with GTP for 1 h in PIPES buffer at 37 °C showed a GTPase activity comparable to that of THD GTP (Supplementary Fig. 25 ), indicating the conversion of THD GTP* into THD GTP . Thus, under the GTP-rich conditions described above, GTP* in CL NC GTP/GTP* is likely replaced with GTP to afford CL NC GTP , which possibly collapses along with the hydrolysis of GTP in a manner analogous to the depolymerization of MT GTP . Of particular importance, CL NC GTP/GTP* remained intact to the treatment with other triphosphates (0.5 mM), such as ATP, cytosine triphosphate CTP, uracil triphosphate UTP (Fig. 4e , Supplementary Figs. 26 and 27 ). Fig. 4: GTP-triggered collapse of CL NC GTP/GTP* . a , b TEM images of CL NC GTP/GTP* after a 100-min incubation with GTP at its concentrations of 0.2 mM ( a ) and 0.5 mM ( b ). c DLS profiles of CL NC GTP/GTP* (8.7 µg ml –1 ) in PIPES buffer after a 100-min incubation with GTP at its concentrations of 0 mM (red), 0.2 mM (orange), 0.5 mM (green), and 1 mM (blue). d GTPase activities of THD GDP (left) and CL NC GTP/GTP* (right) in PIPES buffer. The data was obtained from three biologically independent samples ( n = 3). e DLS profiles of CL NC GTP/GTP* (8.7 µg ml –1 ) in PIPES buffer after a 100-min incubation with 1 mM of ATP (red), CTP (orange), and UTP (green). f TEM image of CL NC GTP/GTP* ⊃ NP Au ([ CL NC GTP/GTP* ] = 13 µg ml –1 , [NP Au ] = 13 pM). g CLSM images of FITC-labeled CL NC GTP/GTP* ⊃ DOX ([ CL NC GTP/GTP* ] = 13 µg ml –1 , [DOX] = 10 µM) incubated without (upper panel) and with (lower panel) 1 mM GTP at 37 °C for 100 min. Micrographs display locations of FITC (i, green) and DOX (ii, red), and their merged images (iii). Scale bars, 2.0 µm. h Fluorescence intensities at 590 nm ( λ ext = 470 nm) of residual DOX obtained after 20, 50, and 100-min incubations of a PIPES solution of CL NC GTP/GTP* ⊃ DOX with 1 mM GTP, followed by ultrafiltration. Red bars represent mean values ± SD from three different samples. Full size image Guest encapsulation into CL NC GTP/GTP* How to stably encapsulate guests inside nanocarriers is one of the important subjects for drug delivery. By using gold nanoparticles (NP Au ; 14 pM, diameter 50 nm) as a guest, we succeeded in obtaining NP Au -encapsulated CL NC GTP/GTP* by adding \({{{\mathrm{Glue}}}}^{{{{\mathrm{CO}}}}_2-}\) (100 µM) to a PIPES buffer solution of a mixture of NS GTP/GTP* (13 µg ml –1 ) and NP Au at 37 °C. After 30-min incubation, the resulting mixture was exposed for 2 min to UV light (300 nm) for crosslinking. Using TEM (Fig. 4f ) and asymmetric field flow fractionation analysis (Supplementary Fig. 28 ), we confirmed that CL NC GTP/GTP* encapsulated NP Au ( CL NC GTP/GTP* ⊃ NP Au ) in its hollow sphere. We also confirmed that CL NC GTP/GTP* , when treated with GTP, indeed released its preloaded guest. For this purpose, we first prepared FITC-labeled THD GDP with a mixture of GTP and GTP* (GTP* content: 83 mol%) in PIPES buffer, and further incubated the resulting fluorescent NS GTP/GTP* with \({{{\mathrm{Glue}}}}^{{{{\mathrm{CO}}}}_2-}\) in the presence of doxorubicin (DOX) for 30 min. Then, the mixture was exposed for 2 min to UV light (300 nm) for transforming NC GTP/GTP* ⊃ DOX into CL NC GTP/GTP* ⊃ DOX, which was confirmed by confocal laser scanning microscopy (CLSM) to carry both FITC and DOX dyes (Supplementary Fig. 29 , green and red, respectively). When CL NC GTP/GTP* ⊃ DOX was incubated with 1 mM GTP in PIPES buffer for 100 min, DOX, as observed by CLSM, became much less fluorescent, indicating the disruption of CL NC GTP/GTP* to release DOX (Fig. 4g , (i)–(iii), lower panel). Upon incubation for 20 min, 50 min, and 100 min, the residues obtained by ultrafiltration (cut-off molecular weight = 5000) of the reaction mixtures contained 73%, 53%, and 21% of the total amount of preloaded DOX, respectively (Fig. 4h ), while in the absence of GTP, DOX was not released (Fig. 4g, (i)–(iii) , upper panel). Intracellular drug delivery with CL NC GTP/GTP* As a proof-of-concept study, we investigated whether FITC-labeled CL NC GTP/GTP* can be taken up by human hepatocellular carcinoma Hep3B cells (Fig. 5a ). The cells were incubated in Eagle’s minimum essential medium (EMEM) containing CL NC GTP/GTP* (0.5 µg ml –1 ) for 2.5 h, rinsed with Dulbecco’s phosphate-buffered saline (D-PBS), and further incubated in EMEM containing 10% fetal bovine serum (FBS) for 1.5 h. CLSM (Fig. 5b (i) , left panel) together with flow cytometry analysis (Fig. 5c ) revealed that most of the cells took up FITC-labeled CL NC GTP/GTP* . Upon subsequent incubation for 21.5 h in EMEM (10% FBS), the entire cytoplasm eventually became fluorescent (Fig. 5b (ii) , right panel) as a possible consequence of the collapse of incorporated CL NC GTP/GTP* . In sharp contrast, FITC-labeled THD GDP and NS GTP/GTP* , the intermediates for constructing CL NC GTP/GTP* , were scarcely taken up into Hep3B cells (Supplementary Figs. 30 and 31 ). 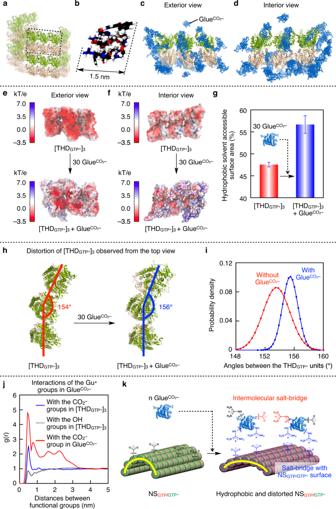Fig. 3: MD simulation of the adhesion events of GlueCO2–onto the surface of THDGTP*. aThree laterally assembled THDGTP*units ([THDGTP*]3) in MTGTP*as a partial model of NS.bAn equilibrated MD snapshot of\({{{\mathrm{Glue}}}}^{{{{\mathrm{CO}}}}_2-}\).c,dThe outer (c) and inner (d) views of [THDGTP*]3hybridized with 30 equivalents of\({{{\mathrm{Glue}}}}^{{{{\mathrm{CO}}}}_2-}\).e,fThe outer (e) and inner (f) views of [THDGTP*]3with its electrostatic surface potential in the absence (upper) and presence (lower) of 30 equivalents of hybridized\({{{\mathrm{Glue}}}}^{{{{\mathrm{CO}}}}_2-}\). Negative and positive potential areas are colored in red and blue, respectively.gThe percentage of hydrophobic solvent-accessible surface area in the absence (47.5 ± 0.5; red) and presence (56.7 ± 2.0; blue) of 30 equivalents of hybridized\({{{\mathrm{Glue}}}}^{{{{\mathrm{CO}}}}_2-}\). Bars represent mean values ± SD from 2000 data points.h,i[THDGTP*]3observed from the top view (h) and its angle distributions (i) in the absence (red) and presence (blue) of 30 equivalents of hybridized\({{{\mathrm{Glue}}}}^{{{{\mathrm{CO}}}}_2-}\).jRadial distribution functions g(r) of the Gu+groups in\({{{\mathrm{Glue}}}}^{{{{\mathrm{CO}}}}_2-}\)with carboxylates (blue) and non-ionic hydroxyl groups (gray) on the [THDGTP*]3surface, and the carboxylate at the focal core of\({{{\mathrm{Glue}}}}^{{{{\mathrm{CO}}}}_2-}\)(red).kSchematic illustration of a possible adhesion event of\({{{\mathrm{Glue}}}}^{{{{\mathrm{CO}}}}_2-}\)onto NSGTP/GTP*and its effects on the features of NSGTP/GTP*. The Gu+groups in\({{{\mathrm{Glue}}}}^{{{{\mathrm{CO}}}}_2-}\)form a salt bridge with carboxylates on the NSGTP/GTP*surface and at the focal core of\({{{\mathrm{Glue}}}}^{{{{\mathrm{CO}}}}_2-}\), and the\({{{\mathrm{Glue}}}}^{{{{\mathrm{CO}}}}_2-}\)-based polymeric network thus formed through this process increases the hydrophobicity of the NSGTP/GTP*surface, making NSGTP/GTP*more flatten. The high intracellular uptake of FITC-labeled CL NC GTP/GTP* is possibly due to a salt-bridge interaction between the Gu + groups in adhering \({{{\mathrm{Glue}}}}^{{{{\mathrm{CO}}}}_2-}\) and cell-surface oxyanionic groups [48] . We confirmed that the intracellular uptake was little affected by the presence of endocytosis inhibitor NaN 3 (ref. 49 ), suggesting that the incorporation of CL NC GTP/GTP* into Hep3B cells was caused via an endocytosis-independent direct pathway (Supplementary Fig. 32 ). For the drug delivery application of CL NC GTP/GTP* , we conducted a cell viability assay with CL NC GTP/GTP* ⊃ DOX. When treated with CL NC GTP/GTP* ⊃ DOX ([ CL NC GTP/GTP* ] = 2.6 µg ml –1 , [DOX] = 2 µM) in EMEM (Fig. 5d ) for 2.5 h, Hep3B cells took up DOX as observed by CLSM after a subsequent incubation in EMEM (10% FBS) for 1.5 h (Fig. 5e (iii) , left panel), and then died within next 21.5 h to form an ill-defined agglomerate (Fig. 5e (iv) , right panel). We also confirmed that Hep3B cells took up a larger amount of DOX in CL NC GTP/GTP* (Fig. 5f , red) than DOX alone (Fig. 5f , orange). Accordingly, CL NC GTP/GTP* ⊃ DOX successfully lowered the cell viability to 30 ± 6% (Fig. 5g , red), whereas that caused by DOX alone was only 48 ± 15% (Fig. 5g , orange). As expected, the cell viability decreased as the concentration of CL NC GTP/GTP* ⊃ DOX was increased (Supplementary Fig. 33 ), while the viability upon incubation with CL NC GTP/GTP* ⊃ DOX did not substantially increase when the incubation time was shortened from 2.5 h to 1.0 h (Supplementary Fig. 34 ). This is likely caused by the GTP-selective collapse of CL NC GTP/GTP* . The intracellular delivery of CL NC GTP/GTP* ⊃ DOX was also successful with other cell lines such as A549 cell and HeLa cell (Supplementary Fig. 35 ). We also confirmed that neither the coexistence of THD GDP nor THD GDP / \({{{\mathrm{Glue}}}}^{{{{\mathrm{CO}}}}_2-}\) enhanced the efficacy of DOX (Supplementary Fig. 36 ). Together with the noncytotoxic nature of CL NC GTP/GTP* (Fig. 5g , green) and its stability in a range of pH at tumor tissue (Fig. 2h ) [50] , these results allow us to expect that CL NC GTP/GTP* may have the potential to deliver preloaded drugs into cancer cells using GTP as an endogenous reporter. Fig. 5: Intracellular drug delivery using CL NC GTP/GTP* . a Schematic illustration of the uptake of FITC-labeled CL NC GTP/GTP* into Hep3B cells. b Bright field (upper row) and CLSM images displaying FITC (middle row, green) in Hep3B cells and their merged images (lower row). The cells were incubated in EMEM containing CL NC GTP/GTP* (0.5 µg ml –1 ) for 2.5 h, rinsed with D-PBS, and further incubated in EMEM (10% FBS) for 1.5 h (i) and 21.5 h (ii). Scale bars, 20 µm. c Flow cytometry profiles showing FITC fluorescence of Hep3B cells ( n > 660) incubated without (blue) and with FITC-labeled CL NC GTP/GTP* for 2.5 h, rinsed with D-PBS, and further incubated in EMEM (10% FBS) for 1.5 h (i, orange) and 21.5 h (ii, green). d Schematic illustration of the cellular uptake of CL NC GTP/GTP* ⊃ DOX. e Bright field (upper row) and CLSM images displaying DOX (middle row, red) in Hep3B cells and their merged images (lower row). The cells were incubated in EMEM containing CL NC GTP/GTP* ⊃ DOX ([ CL NC GTP/GTP* ] = 2.6 µg ml –1 , [DOX] = 2 µM) for 2.5 h, rinsed with D-PBS, and further incubated in EMEM (10% FBS) for 1.5 h (iii) and 21.5 h (iv). Scale bars, 20 µm. f , g Flow cytometry profiles ( f ) showing DOX fluorescence of Hep3B cells ( n > 390) and their normalized viabilities ( g ) determined using Cell Counting Kit-8 ( n = 3). The cells were incubated without (blue) and with DOX (2 µM; orange), and CL NC GTP/GTP* ⊃ DOX ([ CL NC GTP/GTP* ] = 2.6 µg ml –1 , [DOX] = 2 µM; red) for 2.5 h in EMEM, and then rinsed with D-PBS, followed by incubation in EMEM (10% FBS) for 21.5 h. Statistical significance was examined by two-sided Student’s t test (* p = 0.0094 < 0.01). Bars represent mean values ± SD from three different samples. Full size image Here, we have documented the successful reconstitution of MT GTP into a GTP-responsive nanocarrier (Fig. 1 ). MT GTP is depolymerized into THD GDP , which is incubated with a mixture of GTP* and GTP (content of GTP*: 70–85 mol%), thereby facilitating the in situ coassembly of the resulting THD GTP* and THD GTP monomers to form NS GTP/GTP* . 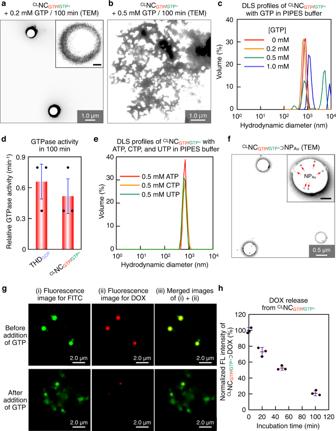Fig. 4: GTP-triggered collapse ofCLNCGTP/GTP*. a,bTEM images ofCLNCGTP/GTP*after a 100-min incubation with GTP at its concentrations of 0.2 mM (a) and 0.5 mM (b).cDLS profiles ofCLNCGTP/GTP*(8.7 µg ml–1) in PIPES buffer after a 100-min incubation with GTP at its concentrations of 0 mM (red), 0.2 mM (orange), 0.5 mM (green), and 1 mM (blue).dGTPase activities of THDGDP(left) andCLNCGTP/GTP*(right) in PIPES buffer. The data was obtained from three biologically independent samples (n= 3).eDLS profiles ofCLNCGTP/GTP*(8.7 µg ml–1) in PIPES buffer after a 100-min incubation with 1 mM of ATP (red), CTP (orange), and UTP (green).fTEM image ofCLNCGTP/GTP*⊃NPAu([CLNCGTP/GTP*] = 13 µg ml–1, [NPAu] = 13 pM).gCLSM images of FITC-labeledCLNCGTP/GTP*⊃DOX ([CLNCGTP/GTP*] = 13 µg ml–1, [DOX] = 10 µM) incubated without (upper panel) and with (lower panel) 1 mM GTP at 37 °C for 100 min. Micrographs display locations of FITC (i, green) and DOX (ii, red), and their merged images (iii). Scale bars, 2.0 µm.hFluorescence intensities at 590 nm (λext= 470 nm) of residual DOX obtained after 20, 50, and 100-min incubations of a PIPES solution ofCLNCGTP/GTP*⊃DOX with 1 mM GTP, followed by ultrafiltration. Red bars represent mean values ± SD from three different samples. 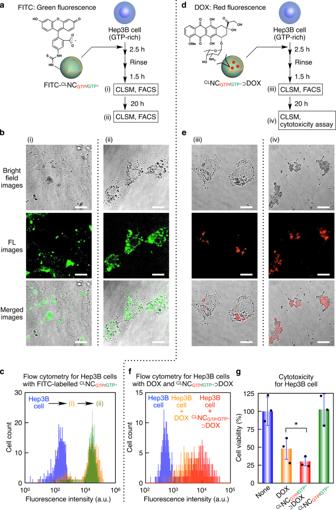Fig. 5: Intracellular drug delivery usingCLNCGTP/GTP*. aSchematic illustration of the uptake of FITC-labeledCLNCGTP/GTP*into Hep3B cells.bBright field (upper row) and CLSM images displaying FITC (middle row, green) in Hep3B cells and their merged images (lower row). The cells were incubated in EMEM containingCLNCGTP/GTP*(0.5 µg ml–1) for 2.5 h, rinsed with D-PBS, and further incubated in EMEM (10% FBS) for 1.5 h (i) and 21.5 h (ii). Scale bars, 20 µm.cFlow cytometry profiles showing FITC fluorescence of Hep3B cells (n> 660) incubated without (blue) and with FITC-labeledCLNCGTP/GTP*for 2.5 h, rinsed with D-PBS, and further incubated in EMEM (10% FBS) for 1.5 h (i, orange) and 21.5 h (ii, green).dSchematic illustration of the cellular uptake ofCLNCGTP/GTP*⊃DOX.eBright field (upper row) and CLSM images displaying DOX (middle row, red) in Hep3B cells and their merged images (lower row). The cells were incubated in EMEM containingCLNCGTP/GTP*⊃DOX ([CLNCGTP/GTP*] = 2.6 µg ml–1, [DOX] = 2 µM) for 2.5 h, rinsed with D-PBS, and further incubated in EMEM (10% FBS) for 1.5 h (iii) and 21.5 h (iv). Scale bars, 20 µm.f,gFlow cytometry profiles (f) showing DOX fluorescence of Hep3B cells (n> 390) and their normalized viabilities (g) determined using Cell Counting Kit-8 (n= 3). The cells were incubated without (blue) and with DOX (2 µM; orange), andCLNCGTP/GTP*⊃DOX ([CLNCGTP/GTP*] = 2.6 µg ml–1, [DOX] = 2 µM; red) for 2.5 h in EMEM, and then rinsed with D-PBS, followed by incubation in EMEM (10% FBS) for 21.5 h. Statistical significance was examined by two-sided Student’sttest (*p= 0.0094 < 0.01). Bars represent mean values ± SD from three different samples. Subsequently, NS GTP/GTP* is treated with molecular glue \({{{\mathrm{Glue}}}}^{{{{\mathrm{CO}}}}_2-}\) to be transformed into spherical NC GTP/GTP* , followed by UV exposure to afford crosslinked CL NC GTP/GTP* capable of stably encapsulating guests (Fig. 2 ). In GTP-rich environments, CL NC GTP/GTP* collapses and releases preloaded guests through the transformation of CL NC GTP/GTP* into CL NC GTP followed by the hydrolysis of its bound GTP into GDP, analogous to the depolymerization of MT GTP (Fig. 4 ). Using CL NC GTP/GTP* , we successfully delivered DOX into cancer cells that overexpress GTP, and caused cell death more efficiently than DOX alone (Fig. 5 ). Most importantly, CL NC GTP/GTP* is a drug carrier that can selectively collapse in response to GTP rather than ATP that is abundant in normal cells. Since cells infected with RNA viruses such as coronavirus produce a large amount of GTP in their self-replication process, GTP is an endogenous reporter for RNA virus-infected cells. In vivo utilization of CL NC GTP/GTP* for curing RNA virus-induced diseases such as COVID-19 is one of the interesting subjects worthy of further investigation. MD simulation was performed using AmberTools 20, GROMACS 2020.5 package, and Visual Molecular Dynamics (VMD) package, and MD simulation methodologies are described in the Supplementary Information . Reconstitution of MT GTP into CL NC GTP/GTP* THD GTP was obtained by purification from porcine brain [51] by two cycles of polymerization and depolymerization in PIPES buffer (100 mM PIPES, 2 mM MgSO 4 , 0.5 mM GTP, 4 µg ml –1 leupeptin, and 0.4 mM PefaBlock, pH 6.8). A solution of THD GTP (5.8 mg ml –1 ) in PIPES buffer (100 mM PIPES, 5 mM MgCl 2 , 2 mM MgSO 4 , 1.5 mM GTP, and 10% DMSO, pH 6.8) was incubated at 37 °C for 30 min to afford MT GTP . The reaction mixture was centrifuged at 17,900 × g for 20 min at 24 °C. The resulting precipitate was dissolved in PIPES buffer (100 mM PIPES, 100 µM MgCl 2 , and 20 µM GDP, pH 6.8) and incubated at 4 °C for 3 h to afford THD GDP [43] . Subsequently, THD GDP (0.3 mg ml –1 ) thus obtained was incubated in PIPES buffer (100 mM PIPES, 1 mM MgCl 2 , 250 µM GTP*, and 50 µM GTP, pH 6.8) at 4 °C for 60 min and then at 37 °C for 30 min to afford NS GTP/GTP* . NS GTP/GTP* (13 µg ml –1 ) was incubated in a solution of \({{{\mathrm{Glue}}}}^{{{{\mathrm{CO}}}}_2-}\) (100 µM) in PIPES buffer (14 mM PIPES, 1 mM MgCl 2 , and 200 µM GTP*, pH 6.8) at 37 °C for 30 min. The reaction mixture was exposed to UV light at 300 nm for 2 min, affording CL NC GTP/GTP* . FITC-labeled NS GTP/GTP* and CL NC GTP/GTP* were prepared using FITC-labeled THD GDP (14% labeling rate) [51] under conditions that were otherwise identical to those listed above. Prior to the NMR measurement of the NS GTP/GTP* sample, unbound GTP and GTP* were removed by centrifugation (286,000 × g ) of the reaction mixture at 37 °C for 60 min. Zeta potentials of NS GTP/GTP* (1.3 µg ml –1 ) and NC GTP/GTP* (1.3 µg ml –1 ) were measured at 37 °C in PIPES buffer. GTP-responsiveness of CL NC GTP/GTP* A solution of CL NC GTP/GTP* (12 µg ml –1 ) in PIPES buffer (9 mM PIPES, 0.9 mM MgCl 2 , and 180 µM GTP*, pH 6.8) was incubated in the presence of GTP (0.1 mM, 0.2 mM, 0.5 mM, and 1 mM), ATP (0.5 mM), CTP (0.5 mM), and UTP (0.5 mM) at 37 °C for 100 min. For the evaluation of the GTP hydrolysis activities of CL NC GTP/GTP* (12 µg ml –1 ) and THD GDP (12 µg ml –1 ), Biomol Green TM reagent (100 µl) was added to the reaction mixtures, incubated for 30 min at room temperature and subjected to electronic absorption spectroscopy at 620 nm. Preparation of CL NC GTP/GTP* ⊃ NP Au CL NC GTP/GTP* ⊃ NP Au was prepared after the incubation of a mixture of NS GTP/GTP* (13 µg ml –1 ), \({{{\mathrm{Glue}}}}^{{{{\mathrm{CO}}}}_2-}\) (100 µM), and gold nanoparticles (NP Au ; 14 pM) in PIPES buffer (14 mM PIPES, 1 mM MgCl 2 , and 200 µM GTP*, pH 6.8) at 37 °C for 30 min, followed by UV irradiation at 300 nm for 2 min. For the asymmetric field flow fractionation analysis, a sample solution of CL NC GTP/GTP* ⊃ NP Au in PIPES buffer was subjected to ultrafiltration (1500 × g ) for 5 min using a regenerated cellulose membrane (cut-off MW = 5000) prior to analysis. PEG-coated NP Au was used to avoid nonspecific adhesion of THD [52] . GTP-triggered release of DOX from CL NC GTP/GTP* CL NC GTP/GTP* ⊃ DOX was prepared after the incubation of a mixture of NS GTP/GTP* (13 µg ml –1 ), \({{{\mathrm{Glue}}}}^{{{{\mathrm{CO}}}}_2-}\) (100 µM), and DOX (10 µM) in PIPES buffer (14 mM PIPES, 1 mM MgCl 2 , and 400 µM GTP*, pH 6.8) at 37 °C for 30 min, followed by UV irradiation at 300 nm for 2 min. The reaction mixture was incubated with GTP (1 mM) at 37 °C for 100 min and then subjected to ultrafiltration (2400 × g ) using a regenerated cellulose membrane (cut-off MW = 5000) for 10 min. The resulting residue was subjected to fluorescence spectroscopy ( λ ext = 470 nm). A reference sample without GTP was likewise prepared. Intracellular delivery Hep3B cells (3.0 × 10 3 cells/well) plated onto an 8-well chambered cover glass were incubated in EMEM containing 10% FBS at 37 °C with 5% CO 2 for 24 h. The cell samples were rinsed twice with D-PBS prior to use. Typically, the cells were treated with FITC-labeled CL NC GTP/GTP* (0.5 µg ml –1 ) and incubated at 37 °C with 5% CO 2 for 2.5 h. Then, the cells were rinsed twice with D-PBS and further incubated at 37 °C for 1.5 h (4-h incubation in total) or 21.5 h (24-h incubation in total) with 5% CO 2 in EMEM containing 10% FBS. Analogous cell samples treated with FITC-labeled THD GDP (0.5 µg ml –1 ), FITC-labeled NS GTP/GTP* (0.5 µg ml –1 ), CL NC GTP/GTP* (0.5 µg ml –1 ) with NaN 3 (5 mM) [49] , CL NC GTP/GTP* ⊃ DOX ([ CL NC GTP/GTP* ] = 2.6 µg ml –1 , [DOX] = 2 µM), CL NC GTP/GTP* (2.6 µg ml –1 ), and DOX (2 µM) were likewise prepared. For a cell viability assay using CL NC GTP/GTP* ⊃ DOX, CL NC GTP/GTP* , and DOX, the cell samples were incubated with Cell Counting Kit-8 reagents (10 µl) for 30 min, and subjected to electronic absorption spectroscopy at 450 nm. Hep3B cell samples treated with Tween 20 (0.2%) were used as a positive control. Statistics and reproducibility All experiments including the preparation of CL NC GTP/GTP* , the investigation of its GTP-responsive collapse, and the intracellular delivery using CL NC GTP/GTP* were performed at least three times to check the reproducibility. Reporting summary Further information on research design is available in the Nature Research Reporting Summary linked to this article.